Drosophilaneuroblasts retain the daughter centrosome During asymmetric mitosis, both in male Drosophila germline stem cells and in mouse embryo neural progenitors, the mother centrosome is retained by the self-renewed cell; hence suggesting that mother centrosome inheritance might contribute to stemness. We test this hypothesis in Drosophila neuroblasts (NBs) tracing photo converted centrioles and a daughter-centriole-specific marker generated by cloning the Drosophila homologue of human Centrobin. Here we show that upon asymmetric mitosis, the mother centrosome is inherited by the differentiating daughter cell. Our results demonstrate maturation-dependent centrosome fate in Drosophila NBs and that the stemness properties of these cells are not linked to mother centrosome inheritance. The correlation between mother versus daughter centrosome segregation and asymmetric cell fate was first documented in Drosophila male germline stem cells (mGSCs), in which the mother centrosome is anchored near the niche and is retained by the stem cell, whereas the daughter centrosome migrates to the opposite side of the cell and is segregated into the differentiating gonial cell after mitosis [1] . More recently, mother centrosome retention has also been demonstrated during asymmetric mitosis in radial glia progenitors in the developing mouse neocortex [2] . In Drosophila mGSCs, the possible functional relevance of such stereotyped centrosome behaviour is still unclear, although tantalizing hypotheses have been put forward [1] , [3] , [4] , [5] . In the developing mouse neocortex, centriole maturation has been shown to be required for maintaining radial glia progenitors [2] . Asymmetric centrosome behaviour has also been documented in Drosophila neuroblasts (NBs) [6] , [7] . NBs are stem-cell-like precursors that generate the fly's central nervous system through a series of asymmetric divisions giving rise to a self-renewed NB and a differentiating ganglion mother cell (GMC), which typically divides only once into a pair of neurons or glia [8] , [9] , [10] . NB asymmetric division is largely driven by cortical polarity. It starts by the apical accumulation of a number of protein complexes including the Par complex (Par-3, Par-6, aPKC) as well as Mushroom body defect, recruited by Partner of Inscuteable, which associates with Gαi, Inscuteable and Par-3 (refs ). Apical complexes control the clustering at the basal cortex of cell fate determinants, such as Numb, Prospero and Brain Tumour, through their adaptor proteins Partner of Numb and Miranda [11] , [16] , [20] , [21] , [22] , [23] , [24] , [25] , [26] , [27] . The apical cortex also controls the orientation of the mitotic spindle along the apico-basal axis, which is essential to position the cytokinesis furrow, such that cleavage segregates the apical and basal sides of the cortex into the newly formed NB and GMC, respectively [28] , [29] , [30] . NB asymmetric division is also controlled by other auxiliary modulators [8] , [9] , [10] . Mosaic clones mutant for any of the known cell fate determinants overgrow in the larval brain and develop as malignant neoplasms upon transplantation into wild-type adult flies, showing that correct execution of the asymmetric division programme in Drosophila NBs is crucial to prevent tumour growth [21] , [22] , [31] , [32] , [33] , [34] , [35] . Centrosomes are important in this process and larval brains that have cells without centrosomes or with more than two centrosomes per cell are highly prone to developing tumours [36] , [37] . NB asymmetry is not limited to cortical polarity at mitosis. Early in interphase, the NB centrosome splits in two, which display significant structural and functional differences [6] , [7] . One of the resulting centrosomes retains most of the pericentriolar material (PCM) and remains at the apical cortex organizing the main microtubule network. The other centrosome has little, if any, PCM and microtubule organizing activity, and migrates extensively across the cytoplasm for most of the interphase [6] , [7] . At mitosis, the apical centrosome is retained by the NB and the other centrosome is inherited by the GMC. Remarkably, at the time of splitting, the GMC-fated centrosome does contain a significant amount of PCM, as revealed by centrosomin fused to GFP which is shed off just before it starts to move [6] . These centrosome asymmetries are thought to have a main role in the orientation of cortical polarity and mitotic spindle alignment [6] , [7] , [38] . Unlike centrioles in vertebrate cells where centriolar satellites, appendages and cartwheel span correlate with centriole maturation [39] , [40] , no ultrastructural dimorphism has been reported between mother and daughter centrioles in Drosophila [41] , [42] . Mother or daughter centriole-specific molecular markers are also lacking in Drosophila . Consequently, it is still unclear if the conspicuously unequal size, activity and fate of Drosophila NBs' centrosomes correlate with centriole maturation. It is also unclear if at the time of splitting each centrosome contains a full diplosome or a single centriole, as it is the case in Drosophila embryos [41] and in some human cell lines [43] , [44] . Here we show by tracing photo-converted centrioles that centrosome splitting occurs before centriole duplication and that the centrosome that loses PCM is motile during interphase. This centrosome is also inherited by the differentiating GMC and contains the mother centriole. We also report the cloning of the Drosophila homologue of Centrobin. In vertebrate cell lines, Centrobin specifically accumulates on the daughter centriole. We find that at the time of centrosome splitting, a yellow fluorescent protein (YFP) fusion to CNB stays on the centrosome that remains at the apical cortex, which is eventually inherited by the NB, and is excluded from the centrosome that breaks away and is fated to the GMC. From these observations, we conclude that centrosome maturation and fate are tightly correlated during asymmetric mitosis in Drosophila NBs, in which the cell that retains stemness inherits the daughter centriole. We also conclude that in spite of the lack of ultrastructural dimorphism, molecular dimorphism exists between mother and daughter Drosophila centrioles. The mother centriole is inherited by the GMC To investigate if mother-versus-daughter centriole differences determine centriole fate during NB asymmetric division, we devised a direct approach based on photo-conversion of a pancentriolar marker in the apical centrosome. There are two expected outcomes of such an experiment ( Fig. 1 ). If at the time of photo-conversion, once the basal centrosome has moved away, the apical centrosome contains two centrioles ( Fig. 1a ), then, in the next cell cycle, both the apical and basal centrosomes will carry the converted signal ( Fig. 1b ). Maturation-dependent centrosome fate will become apparent in the following cycle ( Fig. 1c ) by the consistent segregation of the converted signal, which traces the mother centriole to either the apical centrosome, which is retained in the NB ( Fig. 1c,d ), or the basal centrosome, which is fated to the GMC ( Fig. 1c,d ). Alternatively, if at the time of photo-conversion the apical centrosome contains only one centriole ( Fig. 1e ), the hypothetical maturation-dependent centrosome fate will be revealed in the next cell cycle when, upon centrosome splitting, only the apical or the basal centrosome will carry converted signal ( Fig. 1f ). In such case, the mother centriole will be systematically fated to either the NB ( Fig. 1g ) or the GMC ( Fig. 1g ), respectively. 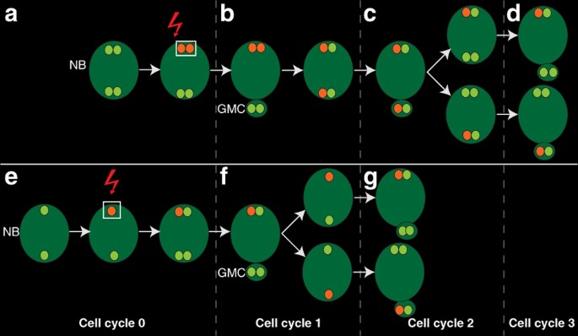Figure 1: Expected outcomes of apical centrosome photo-conversion. Photo-conversion of a centriolar marker in the apical centrosome. (a–d) If at the time of photo-conversion the centrosome contains two centrioles (a, red arrow), the converted signal (red) is retained by the neuroblast (NB), and labels both the apical and basal centrosomes in the next cell cycle (b). In the following cell cycle, consistent segregation of the converted signal to either the apical centrosome (c) or the basal centrosome (c) reveals mother centriole retention by the NB (d) or segregation to the ganglion mother cell (GMC) (d). (e–g) If at the time of photo-conversion the apical centrosome contains only one centriole (e), consistent segregation of the converted signal to the apical or to the basal centrosome in the following cycle (f) demonstrates mother centrosome inheritance by the NB (g) or the GMC (g), respectively. Figure 1: Expected outcomes of apical centrosome photo-conversion. Photo-conversion of a centriolar marker in the apical centrosome. ( a – d ) If at the time of photo-conversion the centrosome contains two centrioles ( a , red arrow), the converted signal (red) is retained by the neuroblast (NB), and labels both the apical and basal centrosomes in the next cell cycle ( b ). In the following cell cycle, consistent segregation of the converted signal to either the apical centrosome ( c ) or the basal centrosome ( c ) reveals mother centriole retention by the NB ( d ) or segregation to the ganglion mother cell (GMC) ( d ). ( e – g ) If at the time of photo-conversion the apical centrosome contains only one centriole ( e ), consistent segregation of the converted signal to the apical or to the basal centrosome in the following cycle ( f ) demonstrates mother centrosome inheritance by the NB ( g ) or the GMC ( g ), respectively. 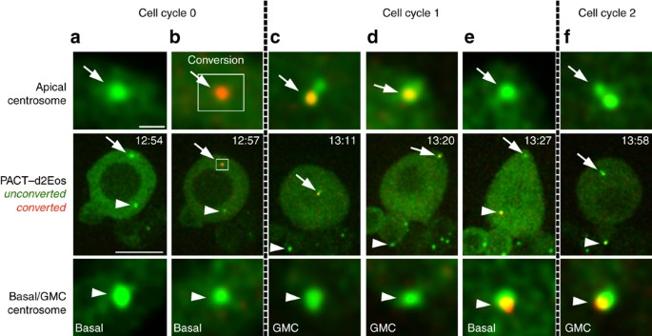Figure 2: The photo-converted mother centriole is inherited by the ganglion mother cell (GMC). Time-lapse series showing a larval neuroblast expressing the photo-convertible pancentriolar marker PACT–d2Eos before (green) and after (red) conversion. Enlarged views of the apical centrosome (arrows) and the corresponding basal or GMC centrosome (arrowheads) are shown in insets above and bellow the central panels. (a) The basal centrosome has migrated away from the apical centrosome. (b) Photo-conversion of the apical centrosome turns fluorescence emission to red, which merged with the green background is seen as orange (cell cycle 0). (c) At mitosis, the apical centrosome, which carries the converted orange signal, stays in the neuroblast (NB). (d) The converted signal is associated with the centrosome that reaches the apical cortex of the NB in early interphase (cell cycle 1). (e) The converted signal, which traces the mother centriole, stays associated with the basal centrosome as it breaks away from the apical centrosome. (f) The basal centrosome carrying the mother centriole is delivered into the GMC at the next mitosis (cell cycle 2). Scale bars equal 10 μm in central panels and 1 μm in upper and lower panels. Time stamp format is hh:mm. Full size image A time-lapse series including the most representative time points of a centrosome photo-conversion experiment using the pancentriolar marker PACT–d2Eos is shown in Figure 2 . After the basal centrosome ( Fig. 2a ) has started to move away from the apical centrosome ( Fig. 2a ), a pulse of 405 nm light is shed on a manually defined rectangular region of interest which overlaps and slightly exceeds the size of the apical centrosome ( Fig. 2b ), causing the photo-conversion of the centriole marker from green to red ( Fig. 2b ). The converted signal remains stably associated with the apical centrosome, which is retained by the NB after the ensuing mitosis ( Fig. 2c ), and migrates to the apical cortex in early interphase ( Fig. 2d ). When the basal centrosome breaks away and starts its characteristic migration through the cytoplasm, the photo-converted signal, which traces the mother centriole, goes with it ( Fig. 2e ) and is subsequently delivered into the GMC at mitosis ( Fig. 2f ). Identical results were obtained in a total of 20 photo-conversion experiments. Figure 2: The photo-converted mother centriole is inherited by the ganglion mother cell (GMC). Time-lapse series showing a larval neuroblast expressing the photo-convertible pancentriolar marker PACT–d2Eos before (green) and after (red) conversion. Enlarged views of the apical centrosome (arrows) and the corresponding basal or GMC centrosome (arrowheads) are shown in insets above and bellow the central panels. ( a ) The basal centrosome has migrated away from the apical centrosome. ( b ) Photo-conversion of the apical centrosome turns fluorescence emission to red, which merged with the green background is seen as orange (cell cycle 0). ( c ) At mitosis, the apical centrosome, which carries the converted orange signal, stays in the neuroblast (NB). ( d ) The converted signal is associated with the centrosome that reaches the apical cortex of the NB in early interphase (cell cycle 1). ( e ) The converted signal, which traces the mother centriole, stays associated with the basal centrosome as it breaks away from the apical centrosome. ( f ) The basal centrosome carrying the mother centriole is delivered into the GMC at the next mitosis (cell cycle 2). Scale bars equal 10 μm in central panels and 1 μm in upper and lower panels. Time stamp format is hh:mm. Full size image Three main conclusions can be derived from these observations. First, at the time when apical and basal centrosomes split in Drosophila NBs, the non-motile apical centrosome contains only one centriole. Second, segregation of mother and daughter centrosomes is highly correlated with asymmetric cell fate. Finally, these results show that NBs retain the daughter rather than the mother centriole. The daughter centriole is inherited by the NB To independently corroborate these conclusions, we decided to circumvent the current lack of molecular markers by cloning the Drosophila homologue of the human daughter-centriole-specific protein Centrobin [45] , [46] . By homology search we identified open reading frame CG5690, predicted to encode a 78.7 kDa protein of 689 aa (Flybase), as the putative Drosophila centrobin ( cnb ) gene. We generated transgenic flies constitutively co-expressing YFP–CNB, and a fusion between mKATE and the pancentriolar marker ASL [47] , and followed the localization of both fluorescent probes in larval NBs. Although, as reported for other centriolar proteins [39] , one or two randomly located YFP–CNB aggregates are often found in these cells ( Fig. 3 ), a clear pattern of YFP–CNB signal segregation emerges. Centrosome-bound YFP–CNB can be observed without interruption from telophase ( Fig. 3a ), up to the time of centrosome splitting, early in the following interphase ( Fig. 3b ). Then, when apical and basal centrosomes break apart, YFP–CNB remains bound to the apical non-motile centrosome ( Fig. 3d ), and cannot be detected over the migrating basal centrosome ( Fig. 3d ). Identical results were obtained in a total of 16 NBs. 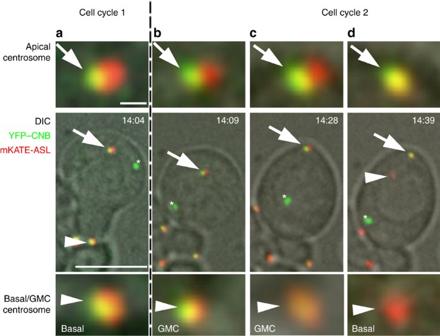Figure 3: The Centrobin-labelled daughter centriole is retained by the apical centrosome. Time-lapse series showing a larval neuroblast co-expressing the daughter centriole marker YFP–CNB (green) and the pancentriolar marker mKATE-ASL (red). Enlarged views of the apical centrosome (arrows) and the corresponding basal or ganglion mother cell (GMC) centrosome (arrowheads) are shown in insets above and below the central panels. (a) YFP–CNB can be detected over both centrosomes at telophase. (b,c) YFP–CNB remains associated with the neuroblast centrosome from cytokinesis (b) to early interphase when the centrosome migrates to the apical cortex (c). (d) When apical and basal centrosomes split apart, YFP–CNB, which traces the daughter centriole, remains on the apical centrosome and cannot be detected in the migrating basal centrosome. One or two YFP–CNB aggregates (asterisks) are often found in NBs expressing mKATE-ASL. Scale bars equal 10 μm in central panels and 1 μm in upper and lower panels. Time stamp format is hh:mm. Figure 3: The Centrobin-labelled daughter centriole is retained by the apical centrosome. Time-lapse series showing a larval neuroblast co-expressing the daughter centriole marker YFP–CNB (green) and the pancentriolar marker mKATE-ASL (red). Enlarged views of the apical centrosome (arrows) and the corresponding basal or ganglion mother cell (GMC) centrosome (arrowheads) are shown in insets above and below the central panels. ( a ) YFP–CNB can be detected over both centrosomes at telophase. ( b , c ) YFP–CNB remains associated with the neuroblast centrosome from cytokinesis ( b ) to early interphase when the centrosome migrates to the apical cortex ( c ). ( d ) When apical and basal centrosomes split apart, YFP–CNB, which traces the daughter centriole, remains on the apical centrosome and cannot be detected in the migrating basal centrosome. One or two YFP–CNB aggregates (asterisks) are often found in NBs expressing mKATE-ASL. Scale bars equal 10 μm in central panels and 1 μm in upper and lower panels. Time stamp format is hh:mm. Full size image Retention of the daughter-centriole marker YFP–CNB by the apical centrosome and the lack of YFP–CNB signal in the motile centrosome corroborates further the conclusions derived from the photo-conversion experiments. In addition, the age-dependent centriole-specific localization of YFP–CNB provides the first instance of molecular asymmetry between mother and daughter Drosophila centrioles. Tracing mother and daughter centrioles with photo-converted PACT–d2Eos and YFP–CNB, respectively, we have shown that apical and basal Drosophila NB centrosomes do not have fully formed diplosomes when they split, and that mother-versus-daughter centriole segregation tightly correlates with cell fate; contrary to what has been generally assumed, the daughter centrosome is fated to be retained by the NB and the mother centrosome is fated to the GMC. The functional relevance of specific centrosome retention by the stem cell in Drosophila remains to be ascertained. Both in mGSCs and in NBs, a microtubule-dependent mechanism hooks one centrosome to the region of the cortex, proximal to the hub in the germ line [1] and apical in NBs [38] ; that is, retained by the stem cell after mitosis. Preferential retention of the mother centrosome in the germ line might therefore simply be the inescapable consequence of carrying more PCM and having greater microtubule-organizing activity [1] . This is less likely in NBs where the daughter centriole is retained, while the mother centriole breaks away carrying little, if any, PCM. That implies the removal of PCM from around the mother centriole and the retention of PCM by the daughter centriole. The shedding of PCM by the GMC-fated centrosome as it splits from the apical centrosome has been previously documented [6] . Precedence for centrosome transmitted cell fate information exist in other species [48] , but not in Drosophila . There are, however, published data on the effect of switching centrosome fate by transient microtubule depolymerization [38] . Upon disassembly of the interphase aster of the NB by treatment with microtubule poisons, the apical centrosome loses connection with the cortex and moves deeper inside the cell so that at mitosis onset, the position of both centrosomes is essentially randomized. Upon recovery of microtubule dynamics, mitosis resumes and asymmetric cell division takes place. In some cases, centrosome fate is switched so that the centrosome originally destined to the GMC is retained by the NB, and vice versa, yet mitosis generates an NB and a GMC that are morphologically normal, strongly suggesting that the identity of the resulting NB and GMC is not severely compromised [38] . It is unknown, however, whether such switch in centriole fate might have long-term developmental consequences. Centriole-maturation-dependent segregation in Drosophila NBs is somewhat reminiscent of spindle pole body (SPB) segregation in budding yeast [49] . Similar to centrioles in animals, the SPB duplicates once per cell cycle. The 'new' SPB remains connected to the 'old' one by the bridge, which is cleaved in S phase. The two SPBs then separate to form the opposite poles of the spindle [50] . In unperturbed cells, the 'old' SPB always migrates into the bud [49] . 'Old' and 'new' SPBs are also functionally and biochemically distinct. For instance, the Bfa1p–Bub2p GTPase-activating protein complex, which is an integral part of the spindle position checkpoint, specifically binds to the 'old' SPB. The SPC inhibits the mitotic exit network) until the nucleus has migrated into the bud [51] , [52] . Also the antigen-presenting cell-related molecule Kar9 localizes only to the 'old' SPB due to the activity of the 'new' SPB-resident Clb4/Cdc28 kinase [53] . Interestingly, SPB fate can also be artificially switched, in which case, Bfa1p still localizes to the SPB that enters the bud independently of whether it is the 'old' or the 'new' [49] , [52] . These data show that in budding yeast biochemical differences between the 'old' and 'new' SPBs are functionally relevant. As in yeast where the 'old' SPB is inherited by the long-lived bud, the mother centriole in Drosophila is inherited in testes by the mGSC, which is the most long-lived of the two mGSC daughters, and in larval brains by the GMC whose daughters outlive the NB. Thus, what appears to be a diametrically different behaviour between mGSCs and NBs using stemness as criteria is consistent, when the expected lifespan of each cell type is considered. During the late stages of the preparation of this manuscript a related paper was published that is fully consistent with our observations [54] . Cloning and transgenesis The PACT domain of Drosophila DPLP [55] was cloned by PCR from pubiPCTGFP (a gift from J. Raff) using the primer pair 5′-gtacggtaccaacatgattgctctgcagaagaaatg-3′ and 5′-gtacctcgagatgatgccgcgcatgcgctctttttg-3′. The PCR product was subcloned into the pcDNA3 Flag1 EosFP tandem vector that contains the tandem dimer version of the photo-convertible EosFP [56] to construct the PACT–d2Eos fusion protein. Using PSI Blast [57] , the Ensemble Genome Browser and InParanoid, we identified CG5690 as the putative Drosophila ortholog of mouse and human centrobin . We obtained the corresponding full-length cDNA, SD06673, from DGRC ( http://dgrc.cgb.indiana.edu ), and fused it to EYFP-C1 (Clontec). We subcloned asl [47] in the pTagFP635-C vector (mKATE, Evrogen). These three fusion constructs were subcloned into the Drosophila pUBq pWRpUbqu transformation vector, and transgenic lines expressing PACT–d2Eos, mKATE-ASL and YFP–CNB under the control of the poly-Ubiquitin promoter were obtained using standard techniques. Microscopy and photo-conversion Primary cultures of larval brain NBs were made by selecting feeding third instar larvae of the appropriate genotype that were surface sterilized in 70% EtOH, rinsed three times in sterile water, and dissected in calcium- and magnesium-free buffer (800 mg of NaCl, 20 mg of KCl, 5 mg of NaH 2 PO 4 , 100 mg of NaHCO 3 and 100 mg of glucose in 100 ml of distilled water) for collagenase (type I, Sigma) treatment (30 min, 0.2 mg ml −1 ). Brains were rinsed three times for 5 min each in Schneider's medium (Gibco), and then they were manually dissociated by repeatedly pipetting the brains up and down in final culture medium [58] using coated yellow tips (Sigmacote, Sigma). Cells were then plated on poly- L -lysin (Sigma)-coated 35 mm glass bottom Fluorodish culture plates (Worldprecision Instruments) and allowed to settle down for 1 h before imaging. Four-dimension time-lapse microscopy was carried out in an ANDOR revolution system equipped with a FRAPPA system and an EMCCD camera on an Olympus IX81 microscope. Photo-conversion was carried out by a pulse of 405 nm laser at 5 μW at the back aperture of a UPLANSAP6 ×100 objective, NA 1.4, and a total pixel dwell time of 900 μs. The photo-converted area was defined by an region of interest surrounding the apical centrosome. Images were recorded before and after conversion using 488 and 561 nm excitation and specific emission filters. No significant red emission was recorded before conversion. How to cite this article: Januschke, J. et al . Drosophila neuroblasts retain the daughter centrosome. Nat. Commun. 2:243 doi: 10.1038/ncomms1245 (2011).